Functional analysis of ade novo GRIN2Amissense mutation associated with early-onset epileptic encephalopathy NMDA receptors (NMDARs), ligand-gated ion channels, play important roles in various neurological disorders, including epilepsy. Here we show the functional analysis of a de novo missense mutation (L812M) in a gene encoding NMDAR subunit GluN2A ( GRIN2A ). The mutation, identified in a patient with early-onset epileptic encephalopathy and profound developmental delay, is located in the linker region between the ligand-binding and transmembrane domains. Electrophysiological recordings revealed that the mutation enhances agonist potency, decreases sensitivity to negative modulators including magnesium, protons and zinc, prolongs the synaptic response time course and increases single-channel open probability. The functional changes of this amino acid apply to all other NMDAR subunits, suggesting an important role of this residue on the function of NMDARs. Taken together, these data suggest that the L812M mutation causes overactivation of NMDARs and drives neuronal hyperexcitability. We hypothesize that this mechanism underlies the patient’s epileptic phenotype as well as cerebral atrophy. N-methyl- d -aspartate receptors (NMDARs) are ligand-gated ion channels that mediate excitatory neurotransmission in the brain. NMDARs are activated following the binding of glutamate and glycine to the GluN1 and GluN2 subunits, respectively. Simultaneous binding of both co-agonists opens a cation-selective pore that results in both depolarization and an increase in the intracellular Ca 2+ concentration. The GluN1 subunit is expressed universally throughout the brain, whereas four different GluN2 subtypes (A–D) have varying temporal and spatial expression in the central nervous system [1] , [2] . The GluN2A and GluN2C subunits are expressed mainly after birth, whereas the expression of GluN2B and GluN2D subunits is highest prenatally and is diminished postnatally in most (but not all) brain regions. NMDARs play important roles in neuronal development, synaptic plasticity, learning and memory, as well as in a wide range of pathological conditions, including epilepsy [3] , [4] . GRIN2A encodes GluN2A and has been genetically associated with autism, schizophrenia, Huntington and Parkinson diseases [5] , [6] , [7] , [8] , [9] , [10] , [11] . Recently, pathogenic mutations in genes encoding NMDARs subunits ( GRIN1 , GRIN2A and GRIN2B ) have been identified in human neurodevelopmental phenotypes, such as, epilepsy, developmental delay or intellectual disability [12] , [13] , [14] , [15] , [16] . Here we present functional analyses for a missense mutation in GRIN2A (GluN2A–L812M) identified in a child with intractable seizures and early-onset epileptic encephalopathy with profound developmental delay. In vitro studies reveal that the L812M mutated receptor has uniquely altered properties that increase NMDAR activity by every measure evaluated, leading to profound hyper-activation of NMDARs, which is almost certainly pathogenic. This residue is closely associated with gating in a conserved region in M4, which is adjacent to the conserved residues SYTANLAAF in the GluN1 M3 transmembrane helix as well as the GluN1 pre-M1 helix. Both the M3 and pre-M1 are proposed to participate in gating [17] . Given the conservation of this residue in all NMDAR subunits, we investigated whether the functional changes of the leucine to methionine mutation transfer to other NMDAR subunits. Our results show that this position is a key structural element of gating that is conserved across the NMDA receptor family. Identification of GRIN2A L812M mutation A six-year-old boy was admitted to the NIH Undiagnosed Diseases Program with a history of intractable infantile-onset epilepsy and profound global developmental delay with no attainment of any milestones, not even head control. At presentation he was having daily, generalized seizures that had been refractory to multiple anti-convulsants including lacosamide, rufinamide and valproic acid. Brain MRI at 6 years of age showed diffuse cerebral parenchymal volume loss and a thin corpus callosum proportionate to the loss of cortical grey matter. There were no dysmorphic features and ophthalmological anomalies. Overall, his clinical history and features were consistent with an early-onset epileptic encephalopathy. Since many early-onset epileptic encephalopathies are due to de novo mutations in ion channels or receptors [18] , [19] , we screened for de novo potentially dominant variants and paired potentially recessive variants with whole-exome sequencing. The only remarkable deleterious variant identified was a heterogeneous, de novo GRIN2A mutation: NCBI nucleotide accession number NM_001134407.1: c.2434C>A (p.Leu812Met, hereafter referred to as L812M), absent in his unaffected sibling as well as in his unaffected parents. The Leu812 residue is highly conserved across vertebrate species and GluN1 and all GluN2 NMDAR subunits ( Fig. 1a ), indicating a possible critical role in NMDAR function. GluN2A–Leu812 resides in the linker region between the lower portion of the agonist-binding domain (S2) and the transmembrane domain (M4) ( Fig. 1a,b ). Using the AMPA receptor structure as a guide [17] , this residue is predicted to reside close enough (within 5 Å) to interact with two potential gating regions in the GluN1 subunit, the M3 transmembrane helix and the pre-M1 helix ( Fig. 1c ). Multiple lines of evidence suggest that a conserved motif (SYTANLAAF) in the M3 transmembrane helix controls gating [17] , [20] , [21] , [22] , [23] , [24] , [25] . Moreover, in AMPA receptors the pre-M1 helix lies in van der Waals contact with the gate and has been suggested to act as a cuff around gating elements that may stabilize the closed state [17] . Interestingly, this site is also a locus for allosteric regulation in NMDA, AMPA and kainate receptors [17] , [26] , [27] , [28] . Our working hypothesis is that the mutation GluN2A–L812M influences a conserved gating control element to both reduce the activation energy to reach the open state and stabilize the open state. A series of electrophysiological experiments were performed to evaluate this hypothesis, and explore the possibility that this mutation could account for this patient’s phenotype. 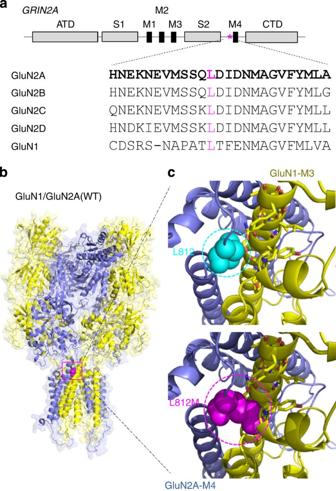Figure 1: Identification of aGRIN2Amissense mutation in a patient with intractable seizures and epileptic encephalopathy. (a) A schematic linear representation of GluN2A. The portions of the polypeptide chain that fold into semiautonomous domains are labelled. The position of the patient’s mutation is indicated by an asterisk. Leu812 is conserved among GluN1 and GluN2 subunits. ATD, amino terminal domain; S1 and S2, agonist-binding domains; M1–4, membrane associated domains 1–4; CTD, carboxy terminal domain. (b) A homology model of the GluN1/GluN2A receptor71built from the GluA2 crystallographic data is shown as ribbon superimposed on a space-filled representation of the receptor. The position of the alteration p.L812M is indicated by magenta colour in the linker region between the ligand-binding and transmembrane domains. (c) An expanded view of the location of residue Leu812 (cyan colour; upper panel) and the possible interaction between L812M (magenta colour; lower panel) and transmembrane domain M3 of GluN1 subunit and a GluN1 pre-M1 helix are predicted from the homomeric GluA2 structure. Figure 1: Identification of a GRIN2A missense mutation in a patient with intractable seizures and epileptic encephalopathy. ( a ) A schematic linear representation of GluN2A. The portions of the polypeptide chain that fold into semiautonomous domains are labelled. The position of the patient’s mutation is indicated by an asterisk. Leu812 is conserved among GluN1 and GluN2 subunits. ATD, amino terminal domain; S1 and S2, agonist-binding domains; M1–4, membrane associated domains 1–4; CTD, carboxy terminal domain. ( b ) A homology model of the GluN1/GluN2A receptor [71] built from the GluA2 crystallographic data is shown as ribbon superimposed on a space-filled representation of the receptor. The position of the alteration p.L812M is indicated by magenta colour in the linker region between the ligand-binding and transmembrane domains. ( c ) An expanded view of the location of residue Leu812 (cyan colour; upper panel) and the possible interaction between L812M (magenta colour; lower panel) and transmembrane domain M3 of GluN1 subunit and a GluN1 pre-M1 helix are predicted from the homomeric GluA2 structure. Full size image GluN2A–L812M enhances agonist potency To investigate whether the mutation GluN2A–L812M influences NMDAR function, site-directed mutagenesis was used to introduce L812M into cDNA encoding the human GluN2A gene product (hereafter hGluN2A). We subsequently expressed wild-type (WT) and mutant hGluN2A with human GluN1 (hGluN1) in Xenopus oocytes and evaluated the concentration–effect curves for glutamate and glycine using a two-electrode voltage-clamp (TEVC). The mutation L812M increased the glutamate potency, as measured by reduction in the half-maximally effective concentration of agonist (EC 50 ) from 3.5 to 0.41 μM ( Fig. 2a , left; Table 1 ). Glycine potency was similarly increased, with the EC 50 decreasing from 1.1 μM in WT to 0.14 μM in mutant receptors ( Fig. 2a , right; Table 1 ). These data showed that the L812M mutation enhanced the potency of glutamate and glycine by eightfold, which will allow the mutant receptor to be activated by much lower concentration of the agonists. 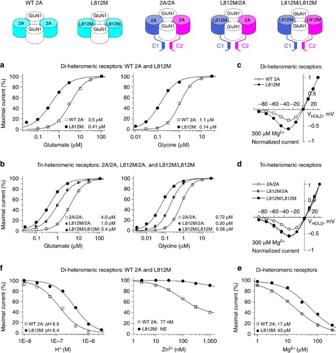Figure 2: The L812M mutation changes the pharmacology of NMDARs. (a,b) Composite concentration–response curves for agonists were determined by TEVC recordings fromXenopusoocytes expressing di-heteromeric GluN1/GluN2A (WT 2A) or GluN1/GluN2A–L812M (L812M) receptors and tri-heteromeric receptors with identity of each GluN2A in the tetrameric complex controlled (for example, GluN1/GluN2A/GluN2A (2A/2A), GluN1/GluN2A–L812M/GluN2A (L812M/2A) and GluN1/GluN2A–L812M/GluN2A–L812M (L812M/L812M)) (see Methods andSupplementary Fig. S2). (a, left) and (b, left) show the composite glutamate (in the presence of 100 μM glycine) concentration–response curves for di-heteromeric receptors and tri-heteromeric receptors. (a, right) and (b, right) show the composite glycine (in the presence of 100 μM glutamate) concentration–response curves for di-heteromeric receptors and tri-heteromeric receptors. (c) Mg2+current–voltage (I–V) curves reveal a decreased Mg2+inhibition for L812M di-heteromeric receptors. (d) Mg2+current–voltage (I–V) curves reveal a dominant decreased Mg2+inhibition in the receptors containing a single copy of L812M. (e) Mg2+concentration–response curves for di-heteromeric receptors are shown. (f) Composite concentration–response curves for proton (left) and zinc (right) inhibition show decreased inhibition of L812M in di-heteromeric receptors. Figure 2: The L812M mutation changes the pharmacology of NMDARs. ( a , b ) Composite concentration–response curves for agonists were determined by TEVC recordings from Xenopus oocytes expressing di-heteromeric GluN1/GluN2A (WT 2A) or GluN1/GluN2A–L812M (L812M) receptors and tri-heteromeric receptors with identity of each GluN2A in the tetrameric complex controlled (for example, GluN1/GluN2A/GluN2A (2A/2A), GluN1/GluN2A–L812M/GluN2A (L812M/2A) and GluN1/GluN2A–L812M/GluN2A–L812M (L812M/L812M)) (see Methods and Supplementary Fig. S2 ). ( a , left) and ( b , left) show the composite glutamate (in the presence of 100 μM glycine) concentration–response curves for di-heteromeric receptors and tri-heteromeric receptors. ( a , right) and ( b , right) show the composite glycine (in the presence of 100 μM glutamate) concentration–response curves for di-heteromeric receptors and tri-heteromeric receptors. ( c ) Mg 2+ current–voltage ( I – V ) curves reveal a decreased Mg 2+ inhibition for L812M di-heteromeric receptors. ( d ) Mg 2+ current–voltage ( I – V ) curves reveal a dominant decreased Mg 2+ inhibition in the receptors containing a single copy of L812M. ( e ) Mg 2+ concentration–response curves for di-heteromeric receptors are shown. ( f ) Composite concentration–response curves for proton (left) and zinc (right) inhibition show decreased inhibition of L812M in di-heteromeric receptors. Full size image Table 1 Summary of pharmacological data for L812M. Full size table Since the L812M mutation of this patient is heterozygous and the tetrameric NMDAR complex contains two GluN2 subunits, we anticipate that some receptors in the patient will contain only a single copy of the mutation. We therefore employed a strategy to control GluN2 trafficking and thus the subunit composition of cell surface NMDARs. We used GluN2A with heterodimeric coiled-coil domains appended to their C termini along with a short dilysine ER retention/retrieval signal comprising KKTN (see Methods). We made a similar pair of constructs harbouring the GluN2A–L812M mutation, which allowed us to express surface receptors with 0, 1 or 2 copies of the mutant GluN2A. We subsequently explored the pharmacology and biophysical properties of these tri-heteromeric receptors. The receptors that contained a single copy of the mutant subunit GluN2A–L812M (referred to as L812M/2A) showed an intermediate increase in glutamate potency (4-fold shift in EC 50 , to 1.0 μM from 4.0 μM for 2A/2A; Fig. 2b , left; Table 1 ) and glycine potency (3.6-fold decrease in EC 50 to 0.20 μM from 0.72 μM for 2A/2A; Fig. 2b , right; Table 1 ). Thus, NMDAR activation was enhanced at lower extracellular concentrations of the agonist even for receptors with a single copy of the mutation. GluN2A–L812M attenuates voltage-dependent Mg 2+ block Voltage-dependent channel block of the NMDAR by extracellular Mg 2+ is an important feature of NMDARs, rendering current flow voltage-dependent [29] , [30] . Two experiments were performed to test whether the GluN2A–L812M alters Mg 2+ inhibition. Evaluation of the current–voltage relationship ( Fig. 2c ; Table 1 ) shows that nearly twice as much current (60 versus 33% for WT) will flow in the mutant compared to WT receptors at negative holding potentials (−30 mV). The concentration–response curves for Mg 2+ block ( Fig. 2e ; Table 1 ) show that this mutation increased the Mg 2+ IC 50 value to 43 μM from 17 μM for WT receptors at the holding potential of −60 mV; similar decreases in potency were observed at other holding potentials (WT versus L812M IC 50 was 455 versus 820 μM at −20 mV, 74 versus 174 μM at −40 mV and 4.7 versus 11 μM at −80 mV). In contrast to the results for agonist potency, a single copy of L812M (L812M/2A) produced a dominant reduction in the Mg 2+ inhibition. The current–voltage relationship ( Fig. 2d ; Table 1 ) shows that more current flows in the single copy of mutant receptors at the negative holding potentials (for example, 55 versus 35% of 2A/2A at −30 mV). A single copy of GluN2A–L812M ( Table 1 ) increased Mg 2+ IC 50 to 38 μM from 15 μM for 2A/2A at the holding potential of −60 mV. As Mg 2+ block occurs deep within the ion channel pore and involves the reentrant pore loops that also control Ca 2+ permeability [3] , [31] , [32] , [33] , we tested whether the L812M mutation alters the calcium permeability. Measurement of the reversal potentials for WT hGluN2A, L812M and WT hGluN2D receptors (as a positive control) in bi-ionic conditions (Ca 2+ or Cs + ) allows the determination of relative Ca 2+ permeability. The data in Supplementary Fig. 1 show that L812M has no detectable effect on the relative Ca 2+ permeability. GluN2A–L812M diminishes negative allosteric regulation Endogenous proton and zinc can inhibit NMDAR function in the central nervous system [3] , and these endogenous ions likely serve as important regulatory mechanisms that limit NMDAR activation. We therefore tested whether the L812M mutation can influence regulation by extracellular zinc or protons. GluN2A–L812M reduced the proton sensitivity, with mutant receptors showing an IC 50 corresponding to pH 6.4, compared with pH 6.9 for WT ( Fig. 2f , left; Table 1 ). The mutation also virtually eliminated high-affinity zinc inhibition for GluN2A–L812M, compared with WT receptors that were inhibited with an IC 50 of 77 nM ( Fig. 2f , right; Table 1 ). Interestingly, a single copy of L812M (L812M/2A) produced a dominant reduction in proton sensitivity with an IC 50 of pH 6.5, compared with pH 6.9 for 2A/2A ( Table 1 ). The single copy of the mutation also produced a dominant decrease in the sensitivity of the receptor to 300 nM extracellular zinc (2A/2A: 34%; L812M/2A: 7.8%; L812M/L812M: 4.8%; Table 1 ). GluN2A–L812M prolongs deactivation time course We next assessed the effect of L812M mutation on the response time course of NMDARs. The deactivation rate following removal from glutamate of NMDARs is thought to control the time course of the NMDAR component of the excitatory postsynaptic current (EPSC) [34] . To evaluate whether the mutation altered the deactivation time course, the current response following glutamate removal was measured using a rapid solution exchange system in whole-cell patch-clamp recordings of WT GluN2A or mutant L812M co-expressed with GluN1 in HEK 293 cells. The deactivation time course of WT 2A following rapid removal of glutamate was fitted by two exponential components with a weighted tau ( τ W ) of 47 ms ( n =11; Fig. 3a ; Table 2 ). The mutant L812M receptors significantly prolonged the glutamate deactivation time course, which was fitted by two exponential components with a τ W of 443 ms ( n =10; Fig. 3a , left; Table 2 ). We also briefly moved the cell into the agonist solution for 3–5 ms (brief application) to mimic synaptic events in the brain. As with the long pulse of agonist, the mutant receptors deactivated with a slower time course compared with WT NMDARs ( τ W 425 versus 44 ms for WT; Fig. 3a , right). The deactivation time course following glycine removal was measured, and could be fitted by two exponential components with a τ W of 63 ms ( n =5; Fig. 3b ; Table 2 ). The mutant GluN2A–L812M receptors showed a slower glycine deactivation time course, which was fitted by two exponential components with a τ W of 691 ms ( n =5; Fig. 3b ; Table 2 ). 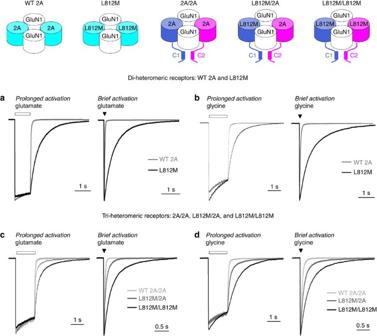Figure 3: The L812M mutation prolongs deactivation time course. (a,b) The L812M mutation prolongs deactivation time course of di-heteromeric GluN2A receptors. (a) The normalized representative current response of di-heteromeric NMDARs (WT 2A and L812M) to 1 mM glutamate (left: long application (1 s) is shown; right: brief application (5 ms); 50 μM glycine in all solutions) (VHOLD−60 mV). L812M (black) prolongs the deactivation time course compared with the WT 2A receptors (grey). (b) The normalized representative current response of di-heteromeric NMDARs to 1 mM glycine is shown (left: long application; right: brief application; 30 μM glutamate in all solutions) (VHOLD−60 mV). (c,d) The L812M mutation prolongs the deactivation time course of tri-heteromeric GluN2A receptors. (c) A representative current response is shown for tri-heteromeric NMDARs with 0, 1 or 2 copies of the L812M mutation in each complex (2A/2A, L812M/2A and L812M/L812M) to 1 mM glutamate (left: long application; right: brief application; 50 μM glycine in all solutions). (d) The normalized representative current response is shown for tri-heteromeric NMDA receptors to 1 mM glycine (left: long application; right: brief application; 30 μM glutamate in all solutions) (VHOLD−60 mV). Figure 3: The L812M mutation prolongs deactivation time course. ( a , b ) The L812M mutation prolongs deactivation time course of di-heteromeric GluN2A receptors. ( a ) The normalized representative current response of di-heteromeric NMDARs (WT 2A and L812M) to 1 mM glutamate (left: long application (1 s) is shown; right: brief application (5 ms); 50 μM glycine in all solutions) ( V HOLD −60 mV). L812M (black) prolongs the deactivation time course compared with the WT 2A receptors (grey). ( b ) The normalized representative current response of di-heteromeric NMDARs to 1 mM glycine is shown (left: long application; right: brief application; 30 μM glutamate in all solutions) ( V HOLD −60 mV). ( c , d ) The L812M mutation prolongs the deactivation time course of tri-heteromeric GluN2A receptors. ( c ) A representative current response is shown for tri-heteromeric NMDARs with 0, 1 or 2 copies of the L812M mutation in each complex (2A/2A, L812M/2A and L812M/L812M) to 1 mM glutamate (left: long application; right: brief application; 50 μM glycine in all solutions). ( d ) The normalized representative current response is shown for tri-heteromeric NMDA receptors to 1 mM glycine (left: long application; right: brief application; 30 μM glutamate in all solutions) ( V HOLD −60 mV). Full size image Table 2 Summary of deactivation time course. Full size table We additionally assessed the time course of deactivation following removal of glutamate or glycine for receptors containing one copy of GluN2A–L812M. As expected, the glutamate and glycine deactivation time constants of receptors with two copies of mutant GluN2A (L812M/L812M) and receptors with no mutation (2A/2A) were comparable to those determined for GluN2A–L812M and WT GluN2A, respectively ( Fig. 3c,d ; Table 2 ). However, the receptors containing a single copy of mutant GluN2A (L812M/2A) showed an intermediate dual exponential glutamate deactivation time course with a τ W of 112 ms ( n =12; Fig. 3c , left; Table 2 ). The NMDAR current response upon briefly moving the cell into the glutamate solution to mimic the synaptic activation showed a similar tendency of the GluN2A–L812M mutation to slow the deactivation time course ( Fig. 3c , right). Furthermore, the receptors containing a single copy of mutant GluN2A (L812M/2A) showed an intermediate slowing of the glycine deactivation time course that could also be described by two exponential components with τ W of 315 ms ( n =7; Fig. 3d , left; Table 2 ), compared with τ W 83 ms for 2A/2A and 784 ms for L812M/L812M. The data from experiments moving the cell briefly into the glycine solution show a similar intermediate effect of the GluN2A–L812M mutation on slowing the glycine deactivation time course ( Fig. 3d , right). These data show that even a single copy of the mutant subunit prolongs the deactivation time course for both agonists, and thus the time course of the NMDAR component of the EPSC. GluN2A–L812M alters single-channel properties We expressed in HEK cells GluN1/GluN2A receptors that contained 0, 1 or 2 copies of the L812M mutation, and excised outside-out patches from these cells. Steady-state single-channel unitary currents were recorded from 2A/2A, L812M/2A and L812M/L812M co-expressed with GluN1 in response to maximally effective concentrations of glutamate and glycine (1,000 μM and 30 μM). Analysis of open time and overall open probability from patches that contained a single active receptor suggested that one copy of the mutant GluN2A subunit within only a single receptor has a dominant effect on open time, shut time and open probability. 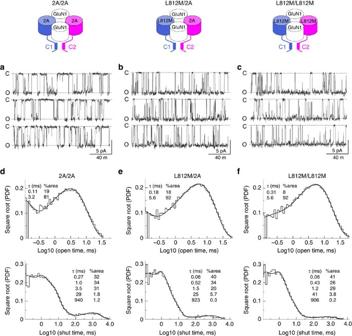Figure 4: The L812M mutation alters the single-channel properties. Steady-state recordings from an outside-out patch containing a single active NMDAR with two WT leucine residues at GluN2A position 812 (2A/2A;a), a single copy of mutation L812M (L812M/2A;b) and two copies of L812M (L812M/L812M;c). Unitary currents were activated in these excised patches by 1 mM glutamate and 50 μM glycine. (d–f) The pooled open duration and shut duration histogram are shown for four single-channel recordings. Open duration histograms were made from 42,302 openings for 2A/2A, 80,303 openings for L812M/2A, 74,138 openings for L812M/L812M. Closed duration histograms were made from 42,299 events for 2A/2A, 80,301 events for L812M/2A, 74,134 events for L812M/L812M. Figure 4a shows 2A/2A single-channel currents that have a complex bursting behaviour with one predominant conductance state (84 pS), and an open probability of 0.21. Open duration and shut duration histograms were fitted with two and five exponential components, respectively. A parallel set of recordings for GluN1 co-expressed with L812M/2A ( Fig. 4b ) and L812M/L812M ( Fig. 4c ) showed identical single-channel conductance (L812M/2A 85pS; L812M/L812M 85pS), but significantly more channel openings with prolonged open periods and shortened shut periods, resulting in an increased open probability. Figure 4d–f and Table 3 summarize the pooled data describing single-channel properties from patches that contained one active channel with GluN2 subunit composition of 2A/2A, L812M/2A and L812M/L812M. Methanethiosulfonate ethylammonium (MTSEA) modification of the A652C mutation in GluN1 SYTANLAAF gating region can lock receptors open [21] , [23] , rendering the degree of potentiation reciprocally related to the open probability prior to MTSEA treatment. Use of this approach to estimate open probability yielded the same result as data from one active channel in excised outside-out patches ( Supplementary Fig. 2 ), confirming a dominant effect on channel gating by a single copy of the mutant receptor. These data indicate that the mutant channels open more often resulting in a profound overactivation of the NMDARs and enhanced neuronal excitability. This situation almost certainly renders neurons vulnerable to excitotoxic neuronal death [35] , [36] . Figure 4: The L812M mutation alters the single-channel properties. Steady-state recordings from an outside-out patch containing a single active NMDAR with two WT leucine residues at GluN2A position 812 (2A/2A; a ), a single copy of mutation L812M (L812M/2A; b ) and two copies of L812M (L812M/L812M; c ). Unitary currents were activated in these excised patches by 1 mM glutamate and 50 μM glycine. ( d – f ) The pooled open duration and shut duration histogram are shown for four single-channel recordings. Open duration histograms were made from 42,302 openings for 2A/2A, 80,303 openings for L812M/2A, 74,138 openings for L812M/L812M. Closed duration histograms were made from 42,299 events for 2A/2A, 80,301 events for L812M/2A, 74,134 events for L812M/L812M. Full size image Table 3 Summary of single-channel properties. Full size table Molecular basis for enhanced NMDA receptor function The residue corresponding to GluN2A–Leu812 is conserved for the GluN1 and GluN2 NMDAR subunits. We hypothesized that this region may play an important role in channel gating [37] , [38] , [39] . To test this idea, we first determined whether changes in agonist potency were associated with the L812M mutation transferred into other GluN subunits at the same position. We substituted Met for Leu in other GluN subunits at the corresponding position, leading to the generation of GluN1–L808M, GluN2B–L813M, GluN2C–L810M, GluN2D–L840M. The potency (EC 50 values) of glutamate and glycine were evaluated for recombinant NMDARs expressed in Xenopus oocytes. The GluN1–L808M mutation co-expressed with GluN2A increased glutamate potency by 9.2-fold (EC 50 : 0.39 versus 3.6 μM for WT 2A) and glycine potency by 9.1-fold (EC 50 : 0.12 versus 1.1 μM for WT) ( Fig. 5a,e ; Table 4 ). GluN1–L808M when co-expressed with GluN2B similarly increased glutamate potency by 6.8-fold ( Fig. 5b ; 0.16 versus 1.3 μM for WT 2B). Likewise, all GluN2 subunits harbouring the L–M mutation showed strongly enhanced potency of both glutamate and glycine ( Fig. 5b–d, f–h ; Table 4 ). These data suggested that the function of the L812 residue is conserved across all GluN1 and GluN2 NMDAR subunits. 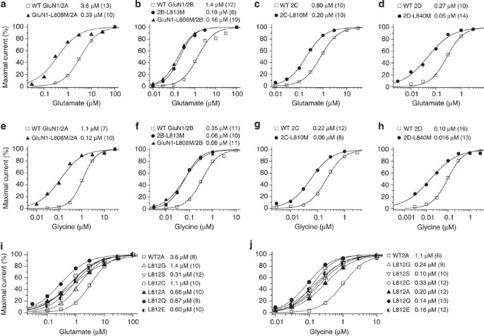Figure 5: The L812M mutation changes agonist potency of other NMDAR subunits. Composite concentration–response curves were determined by TEVC recordings fromXenopusoocytes expressing different GluN subunits-containing receptors (a,e, GluN1/GluN2A and GluN1–L808M/GluN2A;b,f, GluN1/GluN2B, GluN1/GluN2B–L813M and GluN1–L808M/GluN2B;c,g, GluN1/GluN2C and GluN1/GluN2C–L810M;d,h, GluN1/GluN2D and GluN1/GluN2D–L840M). (a–d) show the composite glutamate concentration–response curves determined in the presence of 100 μM glycine. (e–h) show the composite glycine concentration–response curves determined in the presence of 100 μM glutamate. (i,j) show the composite glutamate (i, in the presence of 100 μM glycine) and glycine (j, in the presence of 100 μM glutamate) concentration–response curves of GluN2A–L812G, –L812S, –L812C, –L812A, –L812Q and –L812E. Figure 5: The L812M mutation changes agonist potency of other NMDAR subunits. Composite concentration–response curves were determined by TEVC recordings from Xenopus oocytes expressing different GluN subunits-containing receptors ( a , e , GluN1/GluN2A and GluN1–L808M/GluN2A; b , f , GluN1/GluN2B, GluN1/GluN2B–L813M and GluN1–L808M/GluN2B; c , g , GluN1/GluN2C and GluN1/GluN2C–L810M; d , h , GluN1/GluN2D and GluN1/GluN2D–L840M). ( a – d ) show the composite glutamate concentration–response curves determined in the presence of 100 μM glycine. ( e – h ) show the composite glycine concentration–response curves determined in the presence of 100 μM glutamate. ( i , j ) show the composite glutamate ( i , in the presence of 100 μM glycine) and glycine ( j , in the presence of 100 μM glutamate) concentration–response curves of GluN2A–L812G, –L812S, –L812C, –L812A, –L812Q and –L812E. Full size image Table 4 Summary of agonist EC 50 values for Leu–Met mutations at the position corresponding to GluN2A–Leu812 in all other GluN1 and GluN2 subunits. Full size table We also introduced a series of substitutions (L–G, L–A, L–C, L–S, L–Q and L-E) at this position in GluN2A and assessed the agonist potency. We found increased co-agonist potency in all six mutant receptors ( Fig. 5i,j ; Table 5 ), indicating that the leucine residue at position 812 is critical for NMDAR function. The fact that all perturbations of the side chain tested at this position enhanced NMDAR function may point towards a selective pressure to maintain Leu at this position to limit NMDAR overactivation. Table 5 Summary of agonist EC 50 values for multiple substitutions at GluN2A–Leu812. Full size table Idiopathic epilepsies are considered to be associated with genetic alterations or genetic susceptibility [40] . Several types of epilepsy are due to mutations in single genes, especially those encoding ion channels [40] , [41] . Numerous genes have been associated with early infantile epileptic encephalopathy [42] , [43] . Recently, mutations of GRIN2A have been identified in several cases of early-onset epileptic encephalopathy [12] , [14] , [15] , [16] , [44] . In some of these cases (as in the case we report [45] ), the children did not attain basic milestones. Based on the profound increase in charge transfer predicted for EPSCs from our data as well as the increase in activation by low levels of non-synaptic agonist, we hypothesize that these mutations cause NMDAR hyperactivity and consequently intractable seizures, abnormal development and possible excitotoxic neuronal loss. For this patient, it seems likely that the early-onset epileptic encephalopathy could be due to the reduced block by extracellular Mg 2+ , a >10-fold predicted increase in charge transfer occurring during synaptic transmission, as well as the strong increase in open probability. The greatly increased current flow through GluN2A-containing NMDARs into principle neurons should provide excessive excitatory drive, facilitating or triggering the development of clinically relevant epileptiform activity and perhaps seizures. Compounding this excessive excitatory drive will be activation of NMDARs by low levels of glutamate and/or glycine that would normally be insufficient to induce NMDAR-mediated current flow. Our results with NMDARs that contain a single copy of the mutant receptor show that overactivation does not require two copies of the mutant subunit. This enhanced excitatory drive from all receptors with at least one copy of the mutation could lead to excitotoxic neuronal death, a process long known to occur following overactivation of NMDARs [35] , [36] . This neuronal loss may result in cognitive impairment, motor dysfunction and other neurological problems. Our functional data show that the GluN2A–L812M linker region mutation influences several key features of NMDAR function [37] , [38] , [39] . We interpret all of these effects to be consistent with enhanced gating that could reflect a decrease in the activation energy for pore opening and an increase in stability of the open pore. The pre-M4 linker resides on the immediate extracellular end of M4, placing it between the agonist-binding domain and the transmembrane pore-forming elements. It is therefore a key region for translating the conformational changes induced by agonist binding to opening of the ion channel pore. Previous work with pre-M4 mutations, cross-linking and covalent modification all have suggested a role for the M4 region in gating [37] , [38] , [39] , [46] and in allosteric modulation by the physiologically relevant concentrations of protons [47] . This position has also shown anomalous behaviour in previous studies of covalent modification of Cys residues [37] , [39] . Assuming the NMDARs share similar pore structure as AMPA receptors, examination of the position of Leu812 in GluN2 suggests that it resides within 5 Å of the SYNTANLAAF gating motif in GluN1 M3. The M3 helices are thought to form the helical bundle crossing that occludes ion flow through the pore, and the transmembrane domain M3 is hypothesized to couple agonist binding and channel opening as a transduction element [17] , [21] . M3 residues are also hypothesized to affect cleft closure of the ligand-binding domain, and modification of the M3 conformation by MTSEA (for example, the lurcher site [48] ) influences LBD cleft closure and induces higher agonist potency, slower deactivation time course and decreased sensitivity to competitive antagonists and allosteric modulators (for example, proton inhibition) [20] , [21] , [23] , [49] , [50] . Finally, Leu812 is within 5 Å of the GluN1 pre-M1 helix; both the GluN1 and GluN2 pre-M1 helices lie parallel to the extracellular membrane and are in van der Waals contact with the M3 gate. The pre-M1 region is also a locus for allosteric regulation by exogenous molecules [17] , [28] , [51] . Thus, Leu812 lies at an ideal position to interact with two key elements (the conserved SYTANLAAF gating motif and the pre-M1 helix) hypothesized from structural and functional work to be involved in channel gating. In summary, we present in-depth functional analyses for a unique case of a mutation identified from a patient with intractable seizures, early-onset epileptic encephalopathy associated with progressive cerebral parenchymal volume loss. We report a novel de novo missense mutation in the GRIN2A gene, which dramatically increases the receptor response to agonists, decreases the actions of endogenous negative modulators, increases channel open probability and prolongs deactivation time course and by analogy synaptic duration. The result of this gain-of-function mutation was an increase of over 10-fold in the current mediated by NMDARs, which we predict will contribute to the refractory seizures, cognitive impairment and cortical cell loss in the grey matter. Importantly, this mutation has also allowed the identification of a conserved gating element (that is, Leu812 in GluN2A) that plays a role in the activation of all NMDARs. The proximity of this mutation to a site for allosteric regulation suggests a possible avenue for therapeutic exploration [52] . Moreover, the results suggest that future evaluation of children with refractory seizures and early-onset epileptic encephalopathies might include analysis of the glutamate receptors subunit genes. Whole-exome sequencing DNA was obtained and sequenced based upon clinical protocol 76-HG-0238, ‘Diagnosis and Treatment of Patients with Inborn Errors of Metabolism and other Genetic Disorders’, approved by the NHGRI Institutional Review Board. The parents gave written, informed consent for medical and genetic studies designed to reach diagnoses in the affected children. Exome sequencing was performed using genomic DNA extracted from peripheral blood. In-solution exome capture was performed according to the manufacturer’s protocol using SureSelect Human All Exon Kits (Agilent Technologies, Santa Clara, CA, USA) or the TruSeq Exome Enrichment Kit (Illumina, San Diego, CA, USA). Alignment to the human genome reference sequence (UCSC assembly hg18, NCBI build 36) was carried out using the Efficient Local Alignment of Nucleotide Data algorithm ( Eland , Illumina, Inc). Eland was used in such a way that PE reads were aligned independently, and those that aligned uniquely were grouped into genomic sequence intervals of ~100 kb. Reads that failed to align were binned with their PE mates without Eland using the PE information. Reads that mapped equally well in more than one location were discarded. Crossmatch , a Smith–Waterman-based local alignment algorithm, was used to align binned reads to their respective 100 kb genomic sequence, using the parameters –minscore 21 and –masklevel 0 ( http://www.phrap.org ) [53] . Genotypes were called using a Bayesian genotype caller, Most Probable Genotype (MPG) [54] . To facilitate identification of de novo variants we restricted analysis of exome sequence data to regions of the genome that were routinely well covered and consistently genotyped in 147 exomes from the UDP cohort and 561 exomes from the Clinseq cohort (unaffected individuals). De novo mutations in these regions were identified using a Boolean exclusion filter that selected for variants not present in any other UDP exome and that were at positions for which >50% of the ClinSeq exomes had a successful genotype call. The de novo variants identified were then further filtered to exclude variants present in sequence data derived from unaffected individuals (that is, the ClinSeq cohort or the 1 K genome database of April 2011), in known pseudogenes, or in known artifacts in exome sequencing [55] . Among the variants identified by this process was the c.2434C>A (p.L812M) mutation in exon13 of GRIN2A . Mutagenesis Site-directed mutagenesis was performed using the QuikChange protocol with Pfu DNA polymerase (Stratagene, La Jolla, CA, USA) to replicate the parental strand with desired mismatch incorporated into the primer [23] . Methylated parental DNA template was digested with DpnI. The nicked double-stranded mutant DNA was transformed into TOP10 Competent Cells (Life Tech, Grand Island, NY, USA). The mutations were verified by sequencing through the region of the mutations. The cDNA for WT human NMDA subunit GluN1-1a (hereafter GluN1), GluN2A, GluN2B and GluN2D were in pCI-neo [56] (GenBank accession codes: NP_015566 , NP_000824 , NP_000825 and NP_000827.1 ). The cDNAs for WT rat GluN1 (GenBank accession code: U08261 ), GluN2A (D13211), and GluN2C (M91563) were provided by Drs S. Heinemann (Salk Institute), S. Nakanishi (Osaka Bioscience Institute), and P. Seeburg (University of Heidelberg). The constructs for tri-heteromeric receptors (GluN1/GluN2A/GluN2A, GluN1/GluN2A–L812M/GluN2A and GluN1/GluN2A–L812M/GluN2A–L812M) were prepared by fusing engineered peptide tags, termed C1 and C2, to the C terminus of the rat GluN2A subunit. The two different C1 and C2 tags were composed of a short polypeptide linker containing four repeats of amino acids EAAAK followed by the leucine zipper motifs from GABA B1 or GABA B2 , respectively [57] , and immediately followed by C-terminal di-lysine KKTN endoplasmic reticulum retention/retrieval motifs [58] , [59] , [60] . C1 and C2 were fused to the C terminus of the WT rat GluN2A subunit and the mutant rat GluN2A–L812M to form the following subunits: GluN2A-C1, GluN2A-C2, GluN2A-C1-L812M and GluN2A-C2-L812M. These subunits were then co-expressed with GluN1 to form the following receptors: GluN1/GluN2A-C1/GluN2A-C2 (abbreviated 2A/2A), GluN1/GluN2A-C1-L812M/GluN2A-C2 (abbreviated L812M/2A) and GluN1/GluN2A-C1-L812M/GluN2A-C2-L812M (abbreviated L812M/L812M). The C1 and C2 tags can form a parallel heterodimeric coiled-coil structure, and the KKTN motifs at the distal C termini will localize the subunits in the endoplasmic reticulum unless masked by coiled-coil formation between C1 and C2 (refs 57 , 61 , 62 ). Consequently, the C1 and C2 tags should allow selective surface expression of NMDA receptors composed of two GluN1 subunits, one C1-tagged GluN2A subunit and one C2-tagged GluN2A subunit as evidenced by the control experiments evaluating the escape of non-triheteromeric receptors from the ER retention shown in Supplementary Fig. 3 . This evaluation estimated that <4% of the current responses in the tri-heteromeric experiments were mediated by non-triheteromeric receptors. Two-electrode voltage-clamp recordings cRNA for WT and mutants was synthesized from linearized template of cDNA according to the manufacturer’s specification (Ambion, Austin, TX) and injection of cRNA, as well as two-electrode voltage-clamp recordings from Xenopus laevis oocytes, were performed [63] . Oocytes were obtained from Ecocyte (Austin, TX, USA) and were injected with 5–10 ng cRNAs synthesized in vitro from linearized template cDNA. Following injection, the oocytes were stored at 15–19 °C in Barth’s solution containing (in mM) 88 NaCl, 2.4 NaHCO 3 , 1 KCl, 0.33 Ca(NO 3 ) 2 , 0.41 CaCl 2 , 0.82 MgSO 4 and 5 Tris/HCl (pH 7.4 with NaOH). The ratio of injected di-heteromeric GluN1 to GluN2 cRNA was 1:2. The ratio of injected cRNA for experiments involving tri-heteromeric receptors was 1:6:6 for GluN1:GluN2A-C1:GluN2A-C2, and the cRNA was diluted with RNase-free water to a concentration that would result in ~10 ng total injected cRNA. Voltage-clamp recordings were performed 2–4 days post injection at room temperature (23 °C). The recording solution contained (in mM) 90 NaCl, 1 KCl, 10 HEPES, 0.5 BaCl 2 and 0.01 EDTA (pH 7.4 with NaOH). Solution exchange was computer-controlled through an eight-modular valve positioner (Digital MVP Valve, Hamilton, CT, USA). Voltage and current electrodes were filled with 0.3 and 3.0 M KCl, respectively, and current responses were recorded at a holding potential of −40 mV unless otherwise stated. Data acquisition and voltage control were accomplished with a two-electrode voltage-clamp amplifier (OC725, Warner Instrument, Hamden, CT). Zinc experiments were performed in the tricine solution at (10 mM) pH 7.3. ZnCl 2 solutions (10 mM) were made fresh every day and added directly to the recording solution to obtain the desired nominal Zn 2+ concentration [63] . Glutamate (100 μM) and glycine (100 μM) were used in all oocyte experiments unless otherwise stated. EC 50 values and IC 50 values were obtained by fitting the concentration–response curve with Equation 1 and Equation 2, respectively: where EC 50 is the concentration of agonist that causes a half maximal response, and nH is a slope factor of the response curve. where minimum is the residual percent response in saturating concentration (constrained to >0) of Mg 2+ , protons or zinc, IC 50 is the concentration of antagonist that causes half maximal inhibition, and nH is the slope factor. Preparation and transfection of HEK 293 cells HEK 293 cells (CRL 1573, ATCC, Manassas, VA, USA) or HEK 293 Tet-On Advanced cells (Clontech Laboratories, Mountain View, CA, USA) were plated onto glass coverslips coated in 100 μg ml −1 poly- D -lysine and incubated at 37 °C (5% CO 2 in DMEM/GlutaMax) supplemented with 10% dialyzed fetal bovine serum and 10 μg ml −1 streptomycin. G418 sulphate (150 μg ml −1 ; InvivoGen, San Diego, CA, USA) was added into the medium for HEK 293 Tet-On Advanced cells. HEK 293 cells were co-transfected using the calcium phosphate method [64] with plasmid cDNAs encoding green fluorescent protein (GFP), GluN1 and GluN2A or GluN2A–L812M (ratio was 5:1:1) for di-heteromeric receptor experiments. HEK 293 Tet-On Advanced cells were used for tri-heteromeric receptor experiments and plasmid cDNAs encoding GFP, GluN1, 2A/2A, or L812M/2A or L812M/L812M were transfected at a ratio of 1:1:1:1. In di-heteromeric receptor experiments all receptor subunit cDNA were in the pCI-neo, whereas GluN1 expression was under the control of the Tet-On inducible promoter in the pTRE-tight vector (Clontech Laboratories) in tri-heteromeric receptor experiments.. The mixed plasmid DNA (0.5 μg) was mixed with 6.25 μl of 1 M CaCl 2 , 18.75 μl dH 2 O, 25 μl of 2 × BES solution (50 mM BES, N,N -Bis(2-hydroxyethyl)-2-aminoethanesulfonic acid, N,N -Bis(2-hydroxyethyl)taurine; 280 mM NaCl; 1.5 mM Na 2 HPO4, pH adjusted to 6.95 with HCl) was added, and the mixture was incubated for 5 min at room temperature. Calcium phosphate-DNA solution (50 μl per well) was added dropwise to the plate of cells, and the mixture was swirled gently and incubated for 4 h at 37 °C. After transfection, the cells were incubated overnight post-transfection in standard media supplemented with NMDAR antagonists (200 μM d , L -2-amino-5-phosphonovalerate, 100 μM 7-chlorokynurenic acid and 1,000 μM MgCl 2 ) for both HEK 293 cells and HEK 293 Tet-On Advanced cells. In addition, doxycycline (1–3 μg ml −1 ) was added to the HEK 293 Tet-On Advanced cells to induce expression of GluN1. The following day, ~24 h after transfection, the cells were used for patch-clamp recording (whole-cell voltage-clamp recordings and outside-out single channel recordings). Whole-cell and single-channel voltage-clamp recordings Whole-cell voltage-clamp recordings were performed on transfected HEK 293 cells at −60 mV (23 °C) using an Axopatch 200B amplifier (Molecular Devices, Union City, CA, USA) with micropipettes that contained (in mM) 110 D -gluconate, 110 CsOH, 30 CsCl, 5 HEPES, 4 NaCl, 0.5 CaCl 2 , 2 MgCl 2 , 5 BAPTA, 2 NaATP and 0.3 NaGTP (pH 7.35). Recording electrodes (3–5 ΜΩ) were made from thin-walled glass micropipettes (TW150F-4, World Precision Instruments, Sarasota, FL) pulled using a vertical puller (Narishige P-10, Tokyo, Japan). The external solution contained (in mM) 150 NaCl, 10 HEPES, 30 D -mannitol, 3 KCl, 1.0 CaCl 2 and 0.01 EDTA at 23 °C and pH 7.4. This level of EDTA will chelate with exceptionally high-affinity nM levels of contaminant transition metals (zinc, iron, manganese, and so on) but not significantly alter the extracellular Ca 2+ concentration. Rapid solution exchange with open tip exchange times (<1 ms) for the solutions around the cell was achieved with a two-barrelled theta-glass pipette controlled by a piezoelectric translator (Burleigh Instruments, Newton, NJ, USA) and the data were analysed by ChanneLab (Synaptosoft, Decatur, GA, USA) [65] . Deactivation time course following removal of glutamate was fitted with Equation 3: Single-channel recordings of outside-out patches excised from transfected HEK 293 cells were recorded at −80 mV (digitized at 40 kHz, filtered at 8 kHz) using an Axopatch 200B amplifier at room temperature (23 °C). Recording electrodes were made from thick-walled glass pipettes (G150F-4, Warner Instruments Inc., Hamden, CT, USA) pulled using a vertical puller (Narishige P-10), coated with Sylgard (Dow Corning, Midland, MI, USA) and then fire-polished to 7–9 ΜΩ. The internal solution was the same as that used for the whole-cell voltage-clamp recording. The channel was activated by 1 mM glutamate and 50 μM glycine in an external solution composed of (in mM) 150 NaCl, 10 HEPES, 3 KCl, 0.5 CaCl 2 and 0.01 EDTA at pH 7.4. For analysis, the recordings were pre-filtered at 8 kHz (−3 dB), digitized at 40 kHz and idealized using the Viterbi algorithm in QUB ( http://www.qub.buffalo.edu ) [66] , [67] ; a 100 us open and shut resolution was imposed. Maximum likelihood fitting of open and shut duration histograms was accomplished using ChanneLab (Synaptosoft, Decatur, GA, USA). The single-channel open probability P OPEN was calculated as the ratio of total open duration divided by the sum of total open and closed duration. Evaluation of relative Ca 2+ permeability The relative Ca 2+ permeability (P Ca /P Cs ) was assessed by measuring reversal potential ( V rev ) of WT and mutant NMDARs in bi-ionic conditions (Ca 2+ or Cs + ). The extracellular Ca 2+ solution (1.8 mM ) contained 140 mM NMDG, 10 mM HEPES and 1.8 mM Ca 2+ , adjusted to pH 7.2 by addition of HCl. The extracellular Cs + solution (143 mM) consisted of 140 mM CsCl and 10 mM HEPES, adjusted to pH 7.2 by addition of CsOH. The intracellular recording solution contained (in mM) 125 CsCl, 10 HEPES, 10 EGTA (pH 7.2 by addition of CsOH). The solution was bath-applied by gravity-fed perfusion system and agonists (100 μM glutamate and 100 μM glycine) were applied by fast-perfusion system as for the experiments of deactivation time course. The whole-cell voltage-clamp recordings were performed on HEK 293 cells co-transfected with GluN1, GFP and either WT GluN2A, GluN2A(L812M) or WT GluN2D as a positive control. Current–voltage curves were generated by applying a ramp protocol over −90 to 30 mV (800 ms) after stepping to −90 mV from a holding potential of −60 mV. To minimize voltage changes, a 3 M KCl agarose (0.5%) bridge was used. Liquid junction potential between the extracellular and internal solution were measured (−12.6 mV in 1.8 mM Ca 2+ extracellular solution) and used to correct the holding potential. The current–voltage relationship was fitted by the following Equation 4: The reversal potential was determined as the voltage at which the fitted curve crossed the abscissa. Relative Ca 2+ permeability was calculated with a modified Lewis equation (Equation 5) [68] , [69] , [70] : All reagents were purchased from Sigma. All experiments were performed on two or more separate cell preparations (injected oocytes from different frogs or separate cultures of HEK cells). Data are expressed as mean±s.e.m. and analysed statistically using unpaired t -test and one-way ANOVA with Tukey post hoc test. Significance for all tests was set at P <0.05. Error bars in all figures are s.e.m. How to cite this article: Yuan, H. et al . Functional analysis of a de novo GRIN2A missense mutation associated with early-onset epileptic encephalopathy. Nat. Commun. 5:3251 doi: 10.1038/ncomms4251 (2014).